mTOR coordinates transcriptional programs and mitochondrial metabolism of activated Tregsubsets to protect tissue homeostasis Regulatory T (T reg ) cells derived from the thymus (tT reg ) and periphery (pT reg ) have central and distinct functions in immunosuppression, but mechanisms for the generation and activation of T reg subsets in vivo are unclear. Here, we show that mechanistic target of rapamycin (mTOR) unexpectedly supports the homeostasis and functional activation of tT reg and pT reg cells. mTOR signaling is crucial for programming activated T reg -cell function to protect immune tolerance and tissue homeostasis. T reg -specific deletion of mTOR drives spontaneous effector T-cell activation and inflammation in barrier tissues and is associated with reduction in both thymic-derived effector T reg (eT reg ) and pT reg cells. Mechanistically, mTOR functions downstream of antigenic signals to drive IRF4 expression and mitochondrial metabolism, and accordingly, deletion of mitochondrial transcription factor A (Tfam) severely impairs T reg -cell suppressive function and eT reg -cell generation. Collectively, our results show that mTOR coordinates transcriptional and metabolic programs in activated T reg subsets to mediate tissue homeostasis. Regulatory T (T reg ) cells expressing the transcription factor Foxp3 suppress conventional T-cell responses to establish self-tolerance, prevent autoimmunity, and maintain tissue homeostasis [1] , [2] . Foxp3 deficiency eliminates T reg -cell development and function, leading to autoimmune diseases characterized by excessive T helper 1 (T H 1), T H 2, or T H 17 responses, and germinal center (GC) B-cell reactions driven by T follicular helper (T FH ) cells [3] , [4] , [5] . Thymic-derived T reg (tT reg ) cells exit the thymus and populate peripheral tissues, where resting T reg cells [also called central T reg (cT reg ) cells] are activated in response to antigen and inflammatory cues [6] , [7] , [8] , [9] . These activation signals increase effector molecule expression and induce transcription factors that define the selective suppressive functions and tissue localization of activated T reg cells [also known as effector T reg (eT reg ) cells] [5] , [10] , [11] , [12] , [13] , [14] , [15] . Peripherally-derived T reg (pT reg ) cells are a developmentally distinct population of activated T reg cells that arises from the naive CD4 + T-cell pool and inhibit T H 2 or T H 17 responses at mucosal sites [6] , [16] , [17] , [18] , [19] . The transcription factor interferon regulatory factor 4 (IRF4) is expressed in both eT reg and pT reg cells in vivo and is an essential positive regulator of their homeostasis and function [7] , [15] , [17] , [20] , [21] , [22] . IRF4 expression and function are induced by TCR signals in T reg cells by incompletely understood mechanisms [7] , [8] , [22] . Metabolic rewiring is important for T-cell fate decisions, but the metabolic programs regulating T reg -cell activation and specialization remain uncertain [23] . The activation of the mechanistic target of rapamycin (mTOR) induces metabolic reprogramming necessary for conventional T-cell activation and differentiation [23] , [24] . In contrast, mTOR appears to antagonize T reg -cell differentiation and expansion in vitro and suppressive activity in vivo [23] , [25] , [26] . Mechanistically, inhibition of mTOR upregulates fatty acid oxidation, which supports mitochondrial respiration important for T reg -cell differentiation, proliferation, and survival in vitro [27] , [28] . Moreover, low levels of mTOR activation are needed to prevent excessive glycolysis that can impair T reg -cell survival and lineage stability [23] . Although the prevailing model is that mTOR activation hinders T reg -cell function, T reg cells have higher basal levels of mTORC1 activation than conventional T cells [29] , [30] , which is essential for T reg -cell function in vivo [30] . Thus, mTOR-dependent metabolic programming might have context-dependent roles in different T reg -subsets or under distinct physiological conditions. Here, we show that mTOR orchestrates activation-induced transcriptional and metabolic signatures that are essential for T reg -cell activation and function. We find that either acute or chronic inhibition of mTOR disrupts T reg -cell suppressive activity and leads to uncontrolled conventional T-cell activation. In line with this observation, mucosal CD4 + T-cell responses, including T H 2 responses, are increased when T reg cells lose mTOR, associated with a loss of eT reg and pT reg cells in mucosal sites. Mechanistically, mTOR mediates T reg -cell activation and suppressive activity by promoting IRF4 expression and mitochondrial metabolism. Indeed, disruption of mitochondrial metabolism severely impairs the suppressive function of activated T reg cells and their homeostasis in tissues. Collectively, our results show that mTOR controls peripheral tolerance by integrating transcriptional and metabolic programs critical for the homeostasis and suppressive activity of activated T reg cells. mTOR promotes activated T reg -cell suppressive activity T reg cells activated in vivo have enhanced suppressive activity critical for immune homeostasis [7] , [8] , [31] , [32] , yet the molecular events controlling T reg -cell activation remain to be fully defined. To identify pathways associated with increased suppressive function of T reg cells, we mined a published dataset of activated T reg cells isolated from diphtheria toxin (DT)-treated Foxp3 DTR mice (DTR, diphtheria toxin receptor) [32] . Gene set enrichment analysis (GSEA) revealed that the hallmark mTORC1 and PI3K-Akt-mTOR signaling pathways were among the most significantly (false discovery rate, FDR < 0.05) upregulated gene sets in activated vs. resting T reg cells (Fig. 1a ). Thus, increased T reg -cell suppressive activity is correlated with enhanced mTOR signaling. To rigorously test the function of mTOR for the suppressive activity of activated T reg cells, we activated T reg cells in vitro in the presence or absence of the mTOR inhibitor, PP242. We found that acute inhibition of mTOR diminished the ability of activated T reg cells to suppress conventional T-cell proliferation (Fig. 1b ) and to express the immunosuppressive molecule CTLA4 (Fig. 1c ), indicating a kinase-dependent function of mTOR in T reg -cell function. Accordingly, the suppressive activity of T reg cells isolated from Cd4 Cre Mtor fl/fl mice was dampened (Fig. 1d ). Thus, mTOR is essential for the suppressive function of T reg cells in vitro. Fig. 1 mTOR is essential for activated T reg cell function. a Enrichment plots of the Hallmark mTORC1 (left) and Hallmark PI3K-Akt-mTOR (right) signaling pathways in activated T reg (aT reg ) compared to resting T reg (rT reg ) cells, identified by gene set enrichment analysis (GSEA). The top 20 enriched genes in each pathway (position indicated by the vertical black line) are listed to the right of each plot. b In vitro suppressive activity of T reg cells activated in the presence or absence of PP242. T N : naive CD4 + T cells. c Flow cytometry analysis of CTLA4 expression in T reg cells activated in the presence or absence of PP242. d In vitro suppressive activity of T reg cells isolated from Cd4 Cre Mtor +/+ or +/fl or Cd4 Cre Mtor fl/fl mice. e Representative image of lymphadenopathy in Foxp3 Cre/DTR Mtor fl/fl mice after DT treatment (left). Right, cell numbers of the spleen and peripheral lymph nodes (pLN) of Foxp3 Cre/DTR Mtor +/+ or +/fl or Foxp3 Cre/DTR Mtor fl/fl mice. f Flow cytometry analysis of naive and effector/memory CD4 + Foxp3-YFP − in pLN. g , h Cells from the spleen and pLN of Foxp3 Cre/DTR Mtor +/+ or +/fl or Foxp3 Cre/DTR Mtor fl/fl mice that received DT treatments were stimulated using PMA and ionomycin for 4–5 h. g Flow cytometry analysis of IL-4-producing CD4 + T cells in the spleen and pLN. h Quantification of IFN-γ + CD4 + Foxp3 − and CD8 + T cells or IL-4 + and IL-17A + CD4 + Foxp3 − T cells in the spleen. Error bars show mean ± s.e.m. * P < 0.05; ** P < 0.01; *** P < 0.001; ns, not significant; unpaired, two-tailed Student’s t -test. Data are representative of three ( c ) or four ( e – g ) biological replicates from three ( c ) or two ( e − g ) independent experiments. Data are quantified from three technical replicates representative of three independent experiments ( b , d ) or four or five biological replicates per group as indicated, compiled from two independent experiments ( e , h ). Numbers indicate percentage of cells in gates Full size image To establish a role for mTOR in T reg -cell function in vivo, we generated female Foxp3 Cre/DTR Mtor fl/fl mosaic mice. These mice express a floxed Mtor allele [24] , whose expression can be deleted by Cre recombinase driven under the Foxp3 promoter (denoted as Foxp3 Cre ) [33] , resulting in the deletion of mTOR within T reg cells after they have expressed Foxp3. Acute depletion of DTR-expressing T reg cells with DT forces the remaining Foxp3 Cre -expressing T reg cells to become activated, expand, and control immune homeostasis in adult mice [34] . Upon DT treatment, Foxp3 Cre/DTR Mtor fl/fl mosaic mice, but not their respective Foxp3 Cre/DTR Mtor +/+ or +/fl controls, developed inflammation associated with increased organ size and cell number, especially peripheral lymph nodes (Fig. 1e ). Further, there were increased frequencies of CD44 hi CD62L lo effector/memory CD4 + in the peripheral lymph nodes (Fig. 1f ). After DT treatment, Foxp3 Cre/DTR Mtor fl/fl mice had a profound enrichment for IL-4-producing and small but significant increase in IL-17A-producing, but not IFN-γ-producing, CD4 + T cells in the spleen (Fig. 1g, h ). Similar observations were found in peripheral lymph nodes (Fig. 1g ). Therefore, mTOR signaling is essential for the suppressive function of activated T reg cells, and its acute deletion in T reg cells leads to loss of immune homeostasis and the activation of T H 2, and to a lesser extent, T H 17 cells. T reg cells require mTOR to prevent spontaneous autoimmunity To determine the effects of long-term deletion of Mtor on T reg -cell suppressive function in vivo, we next generated mice bearing a conditional deletion of Mtor within all committed Foxp3 + T reg cells (denoted as Foxp3 Cre Mtor fl/fl mice). As anticipated, Mtor was efficiently deleted within Foxp3-YFP + T reg cells from Foxp3 Cre Mtor fl/fl mice (Supplementary Fig. 1a ). In contrast to their littermate controls that remained healthy, Foxp3 Cre Mtor fl/fl mice developed an early-onset lymphoproliferative and autoimmune disease, indicated by reduced body size and hunched posture, enlargement of peripheral lymphoid organs, and extensive lymphocyte and/or myeloid cell infiltration in multiple organs, such as the skin and lung (Fig. 2a–c ). This disease ultimately led to the early death of Foxp3 Cre Mtor fl/fl mice (Fig. 2d ). These mice had reduced frequencies of CD44 lo CD62L hi naive CD4 + and CD8 + T cells and increased frequencies of CD44 hi CD62L lo effector/memory phenotype CD4 + and CD8 + T cells (Fig. 2e ). There were also significant increases in IFN-γ-, IL-4-, IL-10-, IL-13-, and IL-17A-producing CD4 + T cells and IFN-γ-producing CD8 + T cells in mice with mTOR-deficient T reg cells (Fig. 2f and Supplementary Fig. 1b ). Foxp3 Cre Mtor fl/fl mice had 5–10-fold and 10–15-fold increases in the frequencies of cells producing T H 2- or T H 17-associated cytokines, respectively, while IFN-γ-producing cells were increased by ~5-fold (Supplementary Fig. 1c ). Within T reg cells, the frequency of IFN-γ-producing cells was also increased in Foxp3 Cre Mtor fl/fl mice (Supplementary Fig. 1d ). We also found that the frequencies and total numbers of PD-1 + CXCR5 + T FH cells (Fig. 2g ) and CD95 + GL7 + GC B cells (Fig. 2h ) were increased in Foxp3 Cre Mtor fl/fl mice. We, therefore, performed immunohistochemistry analysis of GCs, B cells, and T cells in whole tissue sections. This analysis revealed that PNA + cells were diffusely distributed in extrafollicular regions, while T and B cells were markedly increased, in mesenteric lymph nodes (Supplementary Fig. 1e ). Foxp3 Cre Rptor fl/fl mice, which have impaired mTORC1 signaling [30] , also had elevated T FH and GC B-cell responses (Supplementary Fig. 1f), indicating that mTORC1 is essential for the T reg -cell-mediated suppression of spontaneous GC reactions. To determine if T FH cells produce elevated levels of IL-4 and/or IL-21 to promote GC reactions [35] , [36] , we isolated CD4 + Foxp3-YFP − CD44 hi CXCR5 − PD-1 − non-T FH cells and CD4 + Foxp3-YFP − CD44 hi CXCR5 + PD-1 + T FH cells from Foxp3 Cre Mtor fl/fl mice and their littermate controls, and measured the expression of Il4 and Il21 . T FH cells from Foxp3 Cre Mtor fl/fl mice had increased expression of Il4 , but not Il21 , while non-T FH cells had increased expression of both Il4 and Il21 (Supplementary Fig. 1g, h ). Thus, constitutive depletion of mTOR revealed its essential role for T reg cell-mediated suppression of conventional T-cell responses in vivo. Fig. 2 Disruption of mTOR in T reg cells results in fatal autoimmunity. a Representative image of 47-day-old Foxp3 Cre Mtor +/fl and Foxp3 Cre Mtor fl/fl littermates. b Representative image of lymphadenopathy in 47-day-old Foxp3 Cre Mtor fl/fl mice (left). Right, cell numbers of the spleen and peripheral lymph nodes (pLN) of Foxp3 Cre Mtor +/+ , Foxp3 Cre Mtor +/fl , or Foxp3 Cre Mtor fl/fl mice. The numbers of mice per group are indicated. c Representative hematoxylin and eosin staining of the indicated tissues from 6-week-old Foxp3 Cre Mtor +/fl and Foxp3 Cre Mtor fl/fl mice. The magnifications are indicated above the respective images for each tissue. d Survival curve of Foxp3 Cre Mtor +/fl and Foxp3 Cre Mtor fl/fl mice. The numbers of mice per group are indicated. e Flow cytometry analysis of naive and effector/memory CD4 + Foxp3-YFP – (depicted as CD4 + ) or CD8 + T-cell populations. f Splenocytes from Foxp3 Cre Mtor +/+ or +/fl and Foxp3 Cre Mtor fl/fl mice were stimulated using PMA and ionomycin for 4–5 h. Cytokine production by CD4 + and CD8 + T cells was assessed by flow cytometry and quantified. g Flow cytometry analysis of PD-1 + CXCR5 + T FH cells. Right, frequency and number of T FH cells in Foxp3 Cre Mtor +/+ or +/fl and Foxp3 Cre Mtor fl/fl mice. h Flow cytometry analysis of CD95 + GL7 + GC B cells. Right, frequency and number of GC B cells in Foxp3 Cre Mtor +/+ or +/fl and Foxp3 Cre Mtor fl/fl mice. Error bars show mean ± s.e.m. * P < 0.05; ** P < 0.01; *** P < 0.001; ns, not significant; unpaired, two-tailed Student’s t -test. Data are representative of at least twelve ( a , b , e ) or three ( c ) biological replicates per group. Data are quantified from the numbers of mice as indicated in the legend key ( b , d ) or from ten or eleven ( f , IFN-γ + and IL-17A + cells from Foxp3 Cre Mtor +/+ or +/fl or Foxp3 Cre Mtor fl/fl mice, respectively), nine or ten ( f , IL-4 + cells from Foxp3 Cre Mtor +/+ or +/fl or Foxp3 Cre Mtor fl/fl mice, respectively), eight ( g ), or nine ( h ) biological replicates per group, compiled from more than eight independent experiments ( f − h ). Numbers indicate percentage of cells in gates Full size image mTOR supports T reg -cell suppression of mucosal T H 2 responses T reg cells regulate T-cell responses important for tissue homeostasis, especially at barrier surfaces like the lung, intestines, and skin [1] , [2] . We found that in the lung of Foxp3 Cre Mtor fl/fl mice, there were respective 5–10-fold and 10–15-fold increases of IL-4- and IL-13-producing CD4 + T cells, while the increases in T H 1 and T H 17 responses were less pronounced (2–3-fold increased) (Fig. 3a and Supplementary Fig. 2a ). T H 2 and T H 17 responses were also more elevated than T H 1 responses in the colon lamina propria (Fig. 3b ). Because we found a consistent increase of T H 2 cytokines in both the lung and colon lamina propria and acute deletion of mTOR led to a profound increase of T H 2 responses (Fig. 1h ), we next performed comprehensive immunohistochemistry analyses of multiple organs in Foxp3 Cre Mtor fl/fl mice. Elevated T H 2 responses are associated with an accumulation of eosinophils, alternatively activated M2 macrophages, and neutrophils in target tissues [16] . Indeed, MBP + eosinophils were increased in the lung (Fig. 3c ), as well as the dermis of the skin (Supplementary Fig. 2b ) of mice-bearing mTOR-deficient T reg cells. Additionally, CD163 + macrophages were expanded, including Ym1 + M2 macrophages present in the alveolar space and interstitium of the lung (Fig. 3d ). Increased M2 macrophage activation was also evident in the skin (Supplementary Fig. 2c ). We also observed an increase of cells positive for iNOS2, which primarily stains for neutrophils, in the lung (Fig. 3e ) and skin (Supplementary Fig. 2d ). T H 2 inflammation is also associated with the accumulation of mucosal mast cells (MMCs) in the intestines [37] . Foxp3 Cre Mtor fl/fl mice had an increase of MCPT1 + interepithelial MMCs and MCPT4 + lamina propria MMCs in the large and small intestines (Fig. 3f ). Altogether, these results underscore an important role for mTOR in mediating T reg -cell-dependent suppression of effector T-cell responses, especially T H 2-associated events, within mucosal tissues. Fig. 3 T reg cells require mTOR for the suppression of mucosal T H 2 responses. a , b Flow cytometry analysis of cytokine-producing CD4 + T cells isolated from the lung ( a ) or colon lamina propria (LP) ( b ) of Foxp3 Cre Mto +/fl or Foxp3 Cre Mtor fl/fl mice. c Representative images of major basic protein (MBP) staining for eosinophils in the lung of Foxp3 Cre Mtor +/fl and Foxp3 Cre Mtor fl/fl mice. d Representative images for M2 macrophages in the lung of Foxp3 Cre Mtor +/fl or Foxp3 Cre Mtor fl/fl mice by CD163 and Ym1 staining. e Representative images for neutrophils, as indicated by inducible nitric oxide synthease 2 (iNOS2) staining, in the lung of Foxp3 Cre Mtor +/fl and Foxp3 Cre Mtor fl/fl mice. f Representative immunohistochemistry of ieMMCs and lpMMCs in the large intestines (left) and small intestines (right) of Foxp3 Cre Mtor fl/+ or Foxp3 Cre Mtor fl/fl mice. Data are representative of four independent experiments ( a , b ) or three biological replicates per group ( c − f ). Numbers indicate percentage of cells in gates Full size image mTOR enforces mucosal tT reg - and pT reg -cell homeostasis Recent work shows that tT reg cells present in tissues exhibit T H 2-biased gene signatures and express transcription factors essential for the suppression of T H 2 responses [12] , [38] , [39] . Additionally, the absence of pT reg cells drives elevated T H 2 responses in mucosal tissues [16] , [17] , [18] . Therefore, we hypothesized that reduced abundance of tT reg and/or pT reg cells might account for increased T H 2 responses in the lung and colon of Foxp3 Cre Mtor fl/fl mice. Neuropilin-1 (Nrp1) and Helios are expressed at higher levels in tT reg than pT reg cells [40] , [41] . We found that there was a significant decrease in the frequency of Nrp1 + tT reg and Nrp1 − pT reg cells in the lung of Foxp3 Cre Mtor fl/fl mice (Fig. 4a ). Helios staining revealed a similar reduction in tT reg and pT reg cells in the lung of Foxp3 Cre Mtor fl/fl mice (Fig. 4b ). We tested if these effects were cell-intrinsic by adoptively transferring an equal ratio of CD45.1 + wild-type bone marrow cells and CD45.2 + Foxp3 Cre Mtor +/fl or Foxp3 Cre Mtor fl/fl bone marrow cells into irradiated Rag1 –/– -recipient mice. This inflammation-free system confirmed that the reduction of these lung T reg -cell populations was cell-intrinsic (Fig. 4c ). We next examined pT reg and tT reg cell populations in the colon lamina propria of Foxp3 Cre Mtor fl/fl mice by staining for either Helios or RORγt, a transcription factor selectively enriched in pT reg cells isolated from the intestines [17] , [19] . Similar to our observations in the lung, pT reg cells, as well as Helios + or RORγt – tT reg cells, were reduced in the colon lamina propria of Foxp3 Cre Mtor fl/fl mice (Fig. 4d, e ). The reduction of RORγt + pT reg cells may also contribute to the increased T H 17 cell activation in the colon lamina propria of Foxp3 Cre Mtor fl/fl mice (Fig. 3b ) [19] . Analysis of Helios + and Helios − T reg -cell populations in the colon lamina propria from mixed bone marrow chimeras verified cell-intrinsic effects (Fig. 4f ). Altogether, these results indicate that the accumulation of mucosal tissue tT reg and pT reg cells is disrupted in the absence of mTOR. Fig. 4 Mucosal tT reg - and pT reg -cell homeostasis is altered in the absence of mTOR. a , b Quantification of the frequencies of Nrp1 + and Nrp1 – ( a ) or Helios + and Helios – T reg cells ( b ) in the lung of Foxp3 Cre Mtor +/+ or +/fl and Foxp3 Cre Mtor fl/fl mice, respectively. c Quantification of the frequencies of Helios + and Helios – T reg cells among the CD45.2 + CD4 + TCRβ + T cells in the lung of mixed bone marrow chimeras. d Quantification of the frequencies of Helios + and Helios – T reg cells in the colon lamina propria of Foxp3 Cre Mtor +/+ or +/fl and Foxp3 Cre Mtor fl/fl mice. e Flow cytometry analysis of Foxp3 vs. RORγt expression (left) and quantification of the frequencies of RORγt + and RORγt – T reg cells (right) in the colon lamina propria of Foxp3 Cre Mtor +/+ or +/fl and Foxp3 Cre Mtor fl/fl mice. f Quantification of the frequencies of Helios + and Helios – T reg cells among the CD45.2 + CD4 + TCRβ + T cells in the colon lamina propria of mixed bone marrow chimeras. g Experimental schematic for in vivo pT reg maintenance assay. h , i Quantification of frequency and/or number of donor-derived Foxp3-YFP + pT reg cells ( h ) or total CD4 + T cells ( i ) in Rag1 –/– mice 4 weeks after adoptive transfer of naive T cells isolated from Foxp3 Cre Mtor +/fl and Foxp3 Cre Mtor fl/fl mice. j Quantification of GATA3 expression in T reg cells stimulated under various conditions (with TGF-β and IL-6 included in all the conditions) for 3 days in the presence or absence of Torin 1. k Quantification of GATA3 + T reg cells (Foxp3 + GATA3 + in CD4 + TCRβ + ) from the colon lamina propria of Foxp3 Cre Mtor +/+ or +/fl and Foxp3 Cre Mtor fl/fl mice. Error bars show mean ± s.e.m. * P < 0.05; ** P < 0.01; *** P < 0.001; ns, not significant; unpaired, two-tailed Student’s t -test. Data are quantified from five ( a , b ), eight ( c ), ten ( d ), eleven ( e ), seven ( f ), three or five ( h , i ; as indicated), three ( j ), or six ( k ) biological replicates, compiled from five ( a , b ), four ( c , f ), eight ( d ), nine ( e ), two ( h , i ), three ( j ), or six ( k ) independent experiments. Numbers indicate percentage of cells in quadrants Full size image To determine the role for mTOR in pT reg -cell maintenance in vivo, we purified naive Foxp3-YFP − CD4 + T cells from either Foxp3 Cre Mtor +/fl or Foxp3 Cre Mtor fl/fl mice and adoptively transferred these cells into Rag1 –/– mice (Fig. 4g ). In this system, naive T cells can acquire Foxp3 expression [42] , and the concomitant expression of the Cre transgene induces Mtor deletion in pT reg cells generated in vivo. The frequency and number of mTOR-deficient pT reg cells were reduced in mesenteric lymph nodes (Fig. 4h ), while the numbers of donor-derived total CD4 + T cells were comparable (Fig. 4i ). These results indicate that mTOR promotes the maintenance of pT reg cells in vivo. Activated T reg cells express GATA3, which is required to suppress T H 2 responses [1] , [2] , [11] , [12] , [16] , [38] . Therefore, we next examined if mTOR regulates GATA3 expression in activated T reg cells. We established an in vitro system where T reg cells from wild-type mice were stimulated with anti-CD3 and anti-CD28 antibodies in the presence of TGF-β and IL-6 to mimic the environmental signals at mucosal sites [1] , [2] , [12] . As expected, compared with IL-2 stimulation, IL-4 strongly upregulated GATA3 expression under these conditions [12] . However, IL-4-induced GATA3 upregulation was diminished upon inhibition of mTOR activity (Fig. 4j ). The frequency of GATA3 + T reg cells was also significantly reduced in the colon lamina propria (Fig. 4k ), a site where these cells are enriched under steady state [11] , [12] . These in vitro and in vivo results highlight the requirement of mTOR signaling for GATA3 expression in T reg cells. mTOR promotes eT reg -cell generation After thymic development, peripheral cT reg cells undergo antigen and inflammation-driven activation and differentiate into eT reg cells that are enriched in tissues, including the lung and colon lamina propria [1] , [2] , [7] , [8] , [21] , [22] . Although eT reg cells are crucial for immune homeostasis, the molecular requirements driving their activation and function are still poorly defined. Our above data indicated that mTOR-deficient tT reg cells were reduced in the lung and colon. Moreover, unbiased GSEA showed that mTORC1 signaling was enriched in CD44 hi CD62L lo eT reg cells compared to CD44 lo CD62L hi cT reg cells (Fig. 5a ). Given these results, we next tested whether mTOR regulates eT reg -cell generation. Because T reg cells isolated from inflammatory environments could undergo secondary phenotypic changes, we analyzed cell-intrinsic effects of mTOR deficiency in cT reg and eT reg cells isolated from healthy, female mosaic mice (designated as Foxp3 Cre/+ ). There was an increase in the frequency but not number of Foxp3-YFP + CD44 lo CD62L hi cT reg cells and a reduction in the frequency and number of Foxp3-YFP + CD44 hi CD62L lo eT reg cells in the spleen of Foxp3 Cre/+ Mtor fl/fl mosaic mice (Fig. 5b ). We also confirmed the reduction of eT reg cells in the spleen of mixed bone marrow chimeras (Supplementary Fig. 3a ). Consistent with elevated mTORC1 signaling in eT reg cells (Fig. 5a ), the frequency and number of eT reg cells were reduced in the absence of Rptor (Supplementary Fig. 3b ). The number of KLRG1 + T reg cells was also reduced in absence of mTOR, consistent with a reduction of eT reg cells (Fig. 5c and Supplementary Fig. 3c ) [9] . The expression of CD25, a marker expressed at higher levels on cT reg cells than eT reg cells [9] , was increased on mTOR-deficient T reg cells (Fig. 5d and Supplementary Fig. 3d ). Moreover, eT reg -cell-associated molecules like ICOS and CTLA4 were expressed at lower levels in the absence of mTOR, while the expression of TIGIT or Foxp3 was equivalent between the control and mTOR-deficient T reg cells (Fig. 5d and Supplementary Fig. 3d ) [1] , [2] , [9] . Activated T reg cells also differentiate into specialized or tissue-resident T reg -cell populations, including CXCR5 + PD1 + Foxp3 + T FR cells that express Bcl6 [5] , [10] , [13] . Both T FR cells and Bcl6 expression were reduced in the absence of mTOR (Fig. 5e and Supplementary Fig. 3e ). Consistent with our earlier analysis of mixed bone marrow chimeras, there was nearly a complete loss of colon T reg cells in Foxp3 Cre Mtor fl/fl mosaic mice (Fig. 5f ). Thus, mTOR is essential for maintaining eT reg cells in vivo. Fig. 5 mTOR is essential for eT reg cell differentiation. a Enrichment plot of the Hallmark mTORC1 pathway activated in eT reg cells compared to cT reg cells, identified by gene set enrichment analysis (GSEA). The top 15 enriched genes (position indicated by the vertical black line) are listed below the plot. b Flow cytometry analysis (left) and quantification of frequencies and cell numbers (right) of CD4 + Foxp3-YFP + CD44 lo CD62L hi cT reg cells and CD4 + Foxp3-YFP + CD44 hi CD62L lo eT reg cells in Foxp3 Cre/+ Mtor +/+ or +/fl and Foxp3 Cre/+ Mtor fl/fl mosaic mice. c Quantification of the number of KLRG1 + T reg cells in the spleen of mixed bone marrow chimeras. d Quantification of CD25, ICOS, CTLA4, TIGIT, and Foxp3 expression in T reg cells from mixed bone marrow chimeras. e Quantification of the frequency of T FR cells (CD4 + Foxp3-YFP + CXCR5 + PD-1 + T reg cells, left) and Bcl6 expression in total Foxp3 + T reg cells (right) in mixed bone marrow chimeras. f Flow cytometry analysis (left) and quantification of the frequency and number (right) of Foxp3-YFP + T reg cells in the colon lamina propria of Foxp3 Cre/+ Mtor +/+ or +/fl and Foxp3 Cre/+ Mtor fl/fl mosaic mice. g Quantification of active caspase-3 in CD45.2 + CD4 + Foxp3-YFP + T reg cells from mixed bone marrow chimeras. h Flow cytometry analysis of CD44 vs. CD62L expression on cT reg cells activated under the indicated conditions for 3 days. US: unstimulated. i Quantification of CD25 and FOXP3 expression in human CD4 + CD25 + CD45RA + CD45RO – naive T reg cells activated for 3 days in the presence or absence of Torin 1 or PP242. Error bars show mean ± s.e.m. * P < 0.05; ** P < 0.01; *** P < 0.001; ns, not significant; unpaired, two-tailed Student’s t -test. Data are representative of at least six ( b ), six ( f ), or three ( h ) biological replicates per group or are quantified from eleven ( b ), fifteen ( c ), seven or eight ( d ; CD45.2 + Foxp3 Cre Mtor +/+ or +/+ chimera or CD45.2 + Foxp3 Cre Mtor +/+ or +/fl mice, respectively; CD25 and Foxp3), ten ( d ; ICOS, CTLA4, and TIGIT; e ), six ( f ), three ( g ), or five ( i ) biological replicates, compiled from seven ( b ), eight ( c ), four ( d , TIGIT; f ), five ( d ; CD25 and Foxp3), six ( d ; ICOS and CTLA4; e ), or two ( g , i ) independent experiments. Numbers indicate percentage of cells in gates Full size image Mechanistically, the loss of eT reg cells in the absence of mTOR could be due to defective survival or reduced activation-induced differentiation. To test the former, we analyzed the expression of active caspase-3 in control and mTOR-deficient T reg cells isolated from mixed bone marrow chimeras and found normal survival of mTOR-deficient T reg cells (Fig. 5g ). Also, the frequency of 7AAD + cells was similar or reduced in purified CD44 lo CD62L hi cT reg cells activated in the presence of the mTOR inhibitors (Supplementary Fig. 3f ), further indicating that mTOR is not essential for cell survival. To test the role of mTOR in activation-induced differentiation, we purified CD44 lo CD62L hi cT reg cells from wild-type mice and activated them for 3 days in the presence or absence of the mTOR inhibitors, Torin 1 and PP242 [43] . We found that cT reg cells differentiation into CD44 hi CD62L lo eT reg -like cells was impaired by mTOR inhibition (Fig. 5h ). Similarly, the frequency of mTOR-deficient T reg cells in the spleen and peripheral lymph nodes of DT-treated Foxp3 Cre/DTR Mtor fl/fl mice was reduced relative to the controls (Supplementary Fig. 3g , left panel), but total numbers of T reg cells were not significantly different (Supplementary Fig. 3g , right panel), likely due to the increased organ size (Fig. 1e ). Thus, mTOR-deficient T reg cells also fail to appropriately respond to activation-induced signals in vivo. We also investigated if these regulatory pathways applied to human cells. In the presence of the mTOR inhibitors, activated human CD45RA hi CD45RO lo naive T reg cells had impaired upregulation of CD25 and FOXP3 (Fig. 5i ), which are expressed more abundantly in human CD45RA lo CD45RO hi activated T reg cells than naive T reg cells [44] . Thus, mTOR activity represents an evolutionarily conserved pathway for driving eT reg -cell generation. mTOR links activation signals to IRF4 upregulation IRF4 is induced by TCR signals to promote eT reg -cell differentiation and regulates T reg -cell-mediated suppression of T H 2 responses in vivo [7] , [8] , [15] , [21] , [22] . To determine if mTOR induces IRF4 expression upon activation, we purified control and mTOR-deficient cT reg cells and activated them for 24 and 48 h before analyzing IRF4 expression by flow cytometry. IRF4 expression was reduced at 24 and 48 h after activation (Fig. 6a ). Acute mTOR inhibition with Torin 1 or PP242 also significantly reduced activation-induced upregulation of IRF4 in cT reg cells (Fig. 6b ). Mechanistically, mTOR controls IRF4 expression at the post-transcriptional level, because cT reg cells activated in the presence of the mTOR inhibitors for 24 or 48 h had increased Irf4 expression compared to the internal controls (Fig. 6c ). To show that the ~20–30% reduction of IRF4 expression was biologically important, we analyzed gene expression profiles in cT reg cells activated in the presence or absence of Torin 1 or PP242. Among the genes that were consistently altered by both inhibitors were 124 IRF4 target genes, including Ccr8 and Eea1 [8] , [15] , [21] , [22] (Fig. 6d ). Also, the loss of IRF4 expression likely accounted for the impairment of mTOR-deficient T reg cells to express ICOS (Fig. 5d and Supplementary Fig. 3d ), which is induced by IRF4-dependent mechanisms to drive eT reg -cell differentiation in vivo [9] , [15] . Altogether, these data indicate that mTOR promotes eT reg -cell differentiation, in part, by modulating IRF4 expression, which also helps explain how T H 2 responses become elevated in Foxp3 Cre Mtor fl/fl mice. Fig. 6 mTOR links activation signals to upregulation of IRF4 expression and downstream targets. a Wild-type (WT) and mTOR-deficient CD4 + Foxp3-YFP + CD44 lo CD62L hi cT reg cells were purified from mixed bone marrow chimeras and activated under the indicated conditions for 24 and 48 h. IRF4 expression was assessed by flow cytometry. b CD4 + Foxp3-YFP + CD44 lo CD62L hi cT reg cells were purified from Foxp3 Cre mice and activated as in a in the presence or absence of Torin 1 and PP242. IRF4 expression was assessed by flow cytometry. c cT reg cells were purified and activated as in b and Irf4 mRNA expression was analyzed by qPCR. d Heat map of IRF4 target genes differentially expressed in resting cT reg cells or cT reg cells activated in the presence of DMSO, Torin 1, or PP242 for 20 h. e Enrichment plot of the Hallmark glycolysis pathway in cT reg cells activated for 20 h in the presence of either Torin 1 or DMSO control, identified by gene set enrichment analysis (GSEA). The top 30 enriched genes (position indicated by the vertical black line) are listed. f Functional enrichment of the IRF4 target genes shown in d . Error bars show mean ± s.e.m. * P < 0.05; ** P < 0.01; *** P < 0.001; ns, not significant; unpaired, two-tailed Student’s t -test. Data are representative of three independent experiments ( b ) or are quantified from five ( a ) and four ( b , c ) biological replicates, compiled from two independent experiments ( a , c ) Full size image mTOR orchestrates mitochondrial metabolism in T reg cells Metabolism is a crucial determinant of T reg -cell biology [23] , but the mechanisms controlling metabolic rewiring required for the function of activated T reg cells are not clear. GSEA showed that cT reg cells upregulated mTORC1 signaling and several metabolic pathways, including glycolysis, upon activation (Supplementary Fig. 4a ), while mTOR inhibitor-treated cT reg cells had a significant downregulation of genes in the glycolytic pathway (Fig. 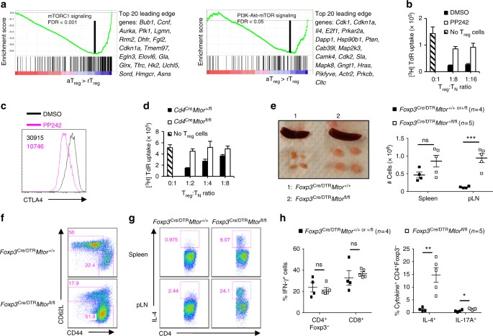Fig. 1 mTOR is essential for activated Tregcell function.aEnrichment plots of the Hallmark mTORC1 (left) and Hallmark PI3K-Akt-mTOR (right) signaling pathways in activated Treg(aTreg) compared to resting Treg(rTreg) cells, identified by gene set enrichment analysis (GSEA). The top 20 enriched genes in each pathway (position indicated by the vertical black line) are listed to the right of each plot.bIn vitro suppressive activity of Tregcells activated in the presence or absence of PP242. TN: naive CD4+T cells.cFlow cytometry analysis of CTLA4 expression in Tregcells activated in the presence or absence of PP242.dIn vitro suppressive activity of Tregcells isolated fromCd4CreMtor+/+ or +/florCd4CreMtorfl/flmice.eRepresentative image of lymphadenopathy inFoxp3Cre/DTRMtorfl/flmice after DT treatment (left). Right, cell numbers of the spleen and peripheral lymph nodes (pLN) ofFoxp3Cre/DTRMtor+/+ or +/florFoxp3Cre/DTRMtorfl/flmice.fFlow cytometry analysis of naive and effector/memory CD4+Foxp3-YFP−in pLN.g,hCells from the spleen and pLN ofFoxp3Cre/DTRMtor+/+ or +/florFoxp3Cre/DTRMtorfl/flmice that received DT treatments were stimulated using PMA and ionomycin for 4–5 h.gFlow cytometry analysis of IL-4-producing CD4+T cells in the spleen and pLN.hQuantification of IFN-γ+CD4+Foxp3−and CD8+T cells or IL-4+and IL-17A+CD4+Foxp3−T cells in the spleen. Error bars show mean ± s.e.m. *P< 0.05; **P< 0.01; ***P< 0.001; ns, not significant; unpaired, two-tailed Student’st-test. Data are representative of three (c) or four (e–g) biological replicates from three (c) or two (e−g) independent experiments. Data are quantified from three technical replicates representative of three independent experiments (b,d) or four or five biological replicates per group as indicated, compiled from two independent experiments (e,h). Numbers indicate percentage of cells in gates 6e and Supplementary Table 1 ), including Hk2 (Fig. 6d ). Because IRF4 also promotes metabolic reprograming of conventional CD4 + and CD8 + T cells [45] , we determined if mTOR signals via IRF4 to regulate T reg -cell metabolism. We performed functional enrichment analysis of IRF4 targets that were differentially expressed in cT reg cells activated in the presence of mTOR inhibitors (Fig. 6d ). This analysis revealed enrichments for glycolytic and nucleotide metabolism and upstream regulators of these pathways, including Myc and mTORC1 [30] , [46] , [47] (Fig. 6f ). Thus, the mTOR-IRF4 axis supports the upregulation of glycolytic and nucleotide metabolism during cT reg -cell activation. Besides glycolysis, cT reg cells upregulated genes in the oxidative phosphorylation pathway in an mTOR-dependent manner (Fig. 7a and Supplementary Table 1 ). Indeed, 366 mitochondrial genes (identified from the MitoCarta 2.0 database [48] ) were differentially expressed in activated cT reg cells (vs. unstimulated cells), and 158 of these genes were mTOR targets (Fig. 7b ). Twenty-one mitochondrial genes were putative IRF4 gene targets (based on IRF4 ChIP-seq analysis [22] ), but only six of these genes were induced upon cT reg -cell activation. Only one of these IRF4 targets ( Mrps28 ) was upregulated in an mTOR-dependent manner during cT reg -cell activation (Fig. 7b ). These data, combined with the functional enrichment analysis above, suggest that mTOR promotes mitochondrial gene expression in a largely IRF4-independent manner. To further test the effects of mTOR on the metabolic pathways, we performed metabolomics profiling using high-resolution mass spectrometry on resting and activated T reg cells. We found that 54 metabolites were differentially expressed between T reg cells activated in the presence of Torin 1 vs. DMSO (Fig. 7c ). For instance, the expression of the TCA cycle intermediates isocitrate/citrate, malate, and succinate and the electron acceptor NAD + were significantly decreased in T reg cells activated in the presence of Torin 1 (Fig. 7c ). 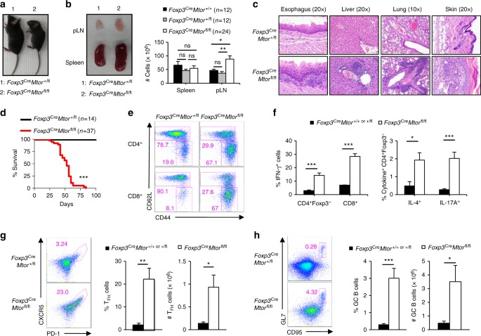Fig. 2 Disruption of mTOR in Tregcells results in fatal autoimmunity.aRepresentative image of 47-day-oldFoxp3CreMtor+/flandFoxp3CreMtorfl/fllittermates.bRepresentative image of lymphadenopathy in 47-day-oldFoxp3CreMtorfl/flmice (left). Right, cell numbers of the spleen and peripheral lymph nodes (pLN) ofFoxp3CreMtor+/+,Foxp3CreMtor+/fl, orFoxp3CreMtorfl/flmice. The numbers of mice per group are indicated.cRepresentative hematoxylin and eosin staining of the indicated tissues from 6-week-oldFoxp3CreMtor+/flandFoxp3CreMtorfl/flmice. The magnifications are indicated above the respective images for each tissue.dSurvival curve ofFoxp3CreMtor+/flandFoxp3CreMtorfl/flmice. The numbers of mice per group are indicated.eFlow cytometry analysis of naive and effector/memory CD4+Foxp3-YFP–(depicted as CD4+) or CD8+T-cell populations.fSplenocytes fromFoxp3CreMtor+/+ or +/flandFoxp3CreMtorfl/flmice were stimulated using PMA and ionomycin for 4–5 h. Cytokine production by CD4+and CD8+T cells was assessed by flow cytometry and quantified.gFlow cytometry analysis of PD-1+CXCR5+TFHcells. Right, frequency and number of TFHcells inFoxp3CreMtor+/+ or +/flandFoxp3CreMtorfl/flmice.hFlow cytometry analysis of CD95+GL7+GC B cells. Right, frequency and number of GC B cells inFoxp3CreMtor+/+ or +/flandFoxp3CreMtorfl/flmice. Error bars show mean ± s.e.m. *P< 0.05; **P< 0.01; ***P< 0.001; ns, not significant; unpaired, two-tailed Student’st-test. Data are representative of at least twelve (a,b,e) or three (c) biological replicates per group. Data are quantified from the numbers of mice as indicated in the legend key (b,d) or from ten or eleven (f, IFN-γ+and IL-17A+cells fromFoxp3CreMtor+/+ or +/florFoxp3CreMtorfl/flmice, respectively), nine or ten (f, IL-4+cells fromFoxp3CreMtor+/+ or +/florFoxp3CreMtorfl/flmice, respectively), eight (g), or nine (h) biological replicates per group, compiled from more than eight independent experiments (f−h). Numbers indicate percentage of cells in gates Unbiased metabolite set enrichment analysis (MSEA) revealed that activated T reg cells significantly upregulated metabolic pathways associated with mitochondria-dependent energy production and the biosynthesis of proteins and nucleotides, such as the citric acid cycle, the mitochondrial electron transport chain, and pyrimidine biosynthesis [49] (Supplementary Fig. 4b ). The upregulation of these mitochondria-related metabolic pathways was impaired when T reg cells were activated in the presence of Torin 1 (Fig. 7d ). Consistent with this observation, T reg cells activated in the presence of Torin 1 had lower mitochondrial membrane potential (TMRM), whereas mitochondria number as indicated by Mitotracker staining was comparable (Fig. 7e ). Thus, mTOR links activation signals to IRF4-dependent and -independent transcriptional programs to induce metabolic reprogramming during T reg -cell activation. Fig. 7 mTOR controls metabolic reprogramming upon T reg -cell activation. a Enrichment plot of the Hallmark oxidative phosphorylation pathway in cT reg cells activated for 20 h in the presence of either Torin 1 or DMSO control, identified by gene set enrichment analysis (GSEA). The top 30 enriched genes (position indicated by the vertical black line) are listed. b Venn-diagram depicting mitochondria-related genes (defined in MitoCarta 2.0 database) that are IRF4 targets (blue circle), or differentially expressed in activated cT reg cells (vs. unstimulated cells; black circle) or activated cT reg cells treated with mTOR inhibitors (vs. those treated with DMSO; red circle). The numbers indicate the shared and independent genes in each category. c Heat map of differentially expressed intracellular metabolites in freshly isolated T reg cells or T reg cells activated for 16 h in the presence of DMSO or Torin 1. d Metabolite set enrichment analysis (MSEA) of KEGG metabolic pathways downregulated in Torin 1-treated activated T reg cells compared to vehicle-treated activated T reg cells. e Flow cytometry of TMRM and Mitotracker staining in T reg cells activated for 20 h in the presence of Torin 1 or vehicle control. Data are representative of three (Mitotracker) or four (TMRM) biological replicates from two (Mitotracker) or three (TMRM) independent experiments ( e ) Full size image Tfam is essential for eT reg -cell homeostasis and function We next genetically defined the importance of mitochondrial metabolism in T reg -cell function in vivo. We conditionally deleted mitochondrial transcription factor A (Tfam), a nuclear-encoded transcription factor essential for efficient electron transport chain activity [50] , [51] , in T reg cells by breeding Foxp3 Cre transgenic mice with mice-bearing floxed alleles for Tfam [51] . Tfam-deficient T reg cells isolated from Foxp3 Cre/+ Tfam fl/fl mosaic mice had comparable mitochondrial content but less mitochondria-derived reactive oxygen species (ROS) (Fig. 8a ), consistent with reduced mitochondrial respiratory chain function. We found that Tfam is critical for T reg -cell function, as Foxp3 Cre Tfam fl/fl mice developed a severe inflammatory disease associated with smaller body size, skin inflammation, alopecia (Fig. 8b ), early lethality (Fig. 8c ), and enlargement of the peripheral lymph nodes (Fig. 8d ). Further, there were increased effector/memory T cells (Fig. 8e ) and significantly enhanced IFN-γ-producing CD8 + T cell and T H 1, T H 2, and T H 17-cell activation (Fig. 8f ) in diseased mice-bearing Tfam-deficient T reg cells. Tfam-deficient T reg cells also had a propensity for increased IFN-γ production (Supplementary Fig. 5a ). Moreover, the frequency and number of T FH cells were increased (Fig. 8g ). Only the frequency, not the number, of GC B cells was increased, likely due to a reduction of total B220 + B cells in Foxp3 Cre Tfam fl/fl mice (Fig. 8h and Supplementary Fig. 5b ). Thus, Tfam deficiency in T reg cells leads to altered immune homeostasis and development of autoimmunity. Fig. 8 Mitochondrial metabolism is critical for T reg -cell function in vivo. a Quantification of Mitotracker (left) and MitoSOX (right) in T reg cells from Foxp3 Cre/+ Tfam +/fl and Foxp3 Cre/+ Tfam fl/fl mosaic mice. b Image of 8-week-old mice. c Survival curve of Foxp3 Cre Tfam +/+ ( n = 14) and Foxp3 Cre Tfam fl/fl mice ( n = 19). d Representative image of lymphadenopathy (left) and cell numbers in the spleen and peripheral lymph nodes (pLN) of Foxp3 Cre Tfam +/fl and Foxp3 Cre Tfam fl/fl mice. e Flow cytometry analysis of naive and effector/memory CD4 + Foxp3-YFP – (depicted as CD4 + ) or CD8 + T cells in Foxp3 Cre Tfam +/fl and Foxp3 Cre Tfam fl/fl mice. f Quantification of cytokine production by CD4 + Foxp3 – and CD8 + T cells. g Flow cytometry analysis (left) and frequency and number (right) of T FH cells. h Flow cytometry analysis (left) and frequency and number (right) of GC B cells. i , j Quantification of frequencies and numbers of cT reg cells and eT reg cells ( i ) or number of KLRG1 + T reg cells ( j ) in the spleen of mixed bone marrow chimeras. k Quantification of ICOS, CTLA4, and TIGIT expression in T reg cells from mixed bone marrow chimeras. l Quantification of the frequency of T FR cells (left) and Bcl6 expression in total Foxp3 + T reg cells (right) in mixed bone marrow chimeras. m , n Quantification of frequency of T reg cells in the colon lamina propria and lung of Foxp3 Cre Tfam +/+ or +/fl or Foxp3 Cre Tfam fl/fl mice ( m ) or mixed bone marrow chimeras ( n ). Error bars show mean ± s.e.m. * P < 0.05; ** P < 0.01; *** P < 0.001; ns, not significant; unpaired, two-tailed Student’s t -test. Data are representative of nine ( b , d , e ), twelve ( g ), or ten ( h ) biological replicates per group, or are quantified from five ( a ), eight or nine ( d , f ; Foxp3 Cre Tfam fl/fl or Foxp3 Cre Tfam +/+ or +/fl mice, respectively), twelve ( g ), ten ( h ), nine or ten ( i − l , n ; CD45.2 + Foxp3 Cre Tfam +/+ chimeras and CD45.2 + Foxp3 Cre Tfam +/fl chimeras, respectively), five ( m , colon), or eight ( m , lung) biological replicates per group, compiled from four ( a ), six ( d , f ), eight ( g ), seven ( h ), four ( i − l , n ), three ( m ; colon), or five ( m ; lung) independent experiments. Numbers indicate percentage of cells in gates Full size image We next analyzed T reg -cell populations in mixed bone marrow chimeras to determine the cell-intrinsic role of Tfam-dependent mitochondrial metabolism in eT reg -cell accumulation and homeostasis. There was a reduction in the frequency and number of CD44 hi CD62L lo eT reg cells (Fig. 8i ) and KLRG1 + T reg cells (Fig. 8j ) in the absence of Tfam. Further, Tfam-deficient T reg cells had reduced expression of ICOS and CTLA4 (Fig. 8k ), but not Foxp3 (Supplementary Fig. 5c ). However, unlike mTOR-deficient T reg cells, CD25 expression was not increased on Tfam-deficient T reg cells (Supplementary Fig. 5c ), and TIGIT expression was reduced (Fig. 8k ). Tfam deficiency also reduced T FR -cell generation and Bcl6 expression (Fig. 8l ). Further, there was a cell-intrinsic reduction of Tfam-deficient T reg cells within the colon lamina propria and the lung (Fig. 8m, n ). Collectively, these results indicate that Tfam-dependent mitochondrial metabolism is critical for the function and homeostasis of activated T reg cells in vivo. Activated tT reg and pT reg cells are crucial for peripheral T-cell tolerance and tissue homeostasis. Here, we show that activated T reg -cell populations have increased mTOR signaling necessary for T reg -cell activation and tissue T reg -cell homeostasis. Mechanistically, mTOR tunes IRF4-dependent transcriptional programming and mitochondrial metabolism. In the absence of mTOR, activated tT reg and pT reg cells are severely decreased in mucosal tissues, associated with excessive T H 2, and to a lesser extent T H 1 and T H 17 responses, and disrupted tissue homeostasis. Further, the homeostasis and suppressive activity of activated T reg cells is impaired by the loss of mitochondrial metabolism and consequently leads to autoimmunity (Supplementary Fig. 5d ). Thus, our data identify and establish a critical mTOR-dependent metabolic node that regulates the homeostasis and suppressive function of activated T reg cells in vivo. TCR-dependent signals coupled with co-stimulation and inflammatory cues drive T reg -cell activation and differentiation into specialized or tissue-resident T reg -cell subsets [1] , [2] , [7] , [8] , [9] , [21] , [22] . Several transcriptional programs are essential for the differentiation and function of activated T reg cells [7] , [20] , [21] , [22] , [43] , [52] , [53] . However, the upstream signaling pathways driving eT reg -cell homeostasis are unknown. Here, we show that activation signals through mTOR are required for T reg -cell activation and function, thereby establishing the first kinase pathway, to our knowledge, that links TCR signals and transcriptional programs necessary for T reg -cell activation. Mechanistically, mTOR promotes the expression of IRF4 and GATA3, transcription factors that are essential for T reg -cell-dependent suppression of T H 2 responses [7] , [11] , [12] , [15] . Moreover, IRF4 also enforces eT reg -cell differentiation and pT reg -cell homeostasis to limit mucosal T H 2 responses [16] , [17] , [20] , [21] , [22] . Therefore, by promoting the expression of IRF4 and GATA3, mTOR maintains activated T reg -cell populations that facilitate tissue homeostasis. The mTOR-dependent induction of IRF4 expression in cT reg cells was not transcriptionally regulated, and, in conventional CD4 + T cells [54] , occurs independently of the mTOR-4EBP1 translation axis. Therefore, mTOR likely regulates IRF4 expression at the post-translational level, such as via SUMOlyation [55] . A key question that remains is, why are mucosal tissues more sensitive to the upregulation of T H 2 responses than secondary lymphoid organs in mice-bearing mTOR-deficient T reg cells? One possibility is that these sites are enriched for activated tT reg - and pT reg -cell populations and hence their loss more readily increases T H 2 responses at these sites than in the peripheral lymphoid organs [1] , [2] , [56] . Further, recent work shows that tissue T reg cells express high levels of ST2 (IL-33 receptor) [38] , [39] , which induces GATA3 activation that biases T reg cells toward the T H 2 suppressive program [39] . Thus, mTOR deficiency and other conditions that decrease GATA3 expression will impair this feed forward loop and disrupt T H 2-like T reg -cell suppressive responses. Metabolic reprogramming contributes to cell fate decisions. However, the metabolic programs promoting the homeostasis and function of activated T reg cells are not completely understood [23] . Despite the previous work suggesting an inhibitory role of mTOR for mitochondrial oxidative metabolism in induced T reg cells in vitro [27] , we show here that mitochondrial metabolism is highly induced during T reg -cell activation in an mTOR-dependent manner, and is essential for activated T reg -cell function and tissue homeostasis in vivo. Indeed, T reg -specific deletion of Tfam impairs T reg -cell function, leading to the hyperactivation of conventional T cells and autoimmunity. Mechanistically, mitochondrial metabolism could affect eT reg -cell proliferation or survival within tissues as has been reported in vitro [27] , [28] . Of note, Raptor-deficient T reg cells have reduced mitochondria-related gene expression [30] , and Foxp3 Cre Tfam fl/fl and Foxp3 Cre Rptor fl/fl mice have similar elevations in activated T-cell responses, disease pathologies, and survival kinetics [30] . Additionally, deficiency of Tfam and Raptor impairs T FR cell accumulation [57] . Thus, our data suggest a key role for Raptor-mTORC1-induced mitochondrial metabolism in establishing the fate and function of activated T reg cells in different microenvironments. T reg cells must adapt to different environmental cues to acquire unique suppressive functions, and the appropriate balance of mTOR and metabolic signaling appears to be linked to this process. Inactivation of mTORC1 alone or combined with mTORC2 disrupts T reg -cell suppressive activity [30] ; however, whether mTORC1-independent functions of Raptor [58] or Raptor/Rictor-independent mTOR complexes play roles in T reg -cell biology remained unclear. Our results here suggest that mTOR does act through Raptor and Rictor to promote T reg -cell function. Compared to Raptor deficiency alone, loss of mTOR or Raptor and Rictor in T reg cells leads to similar extensions in lifespan [30] , which may be due to more limited tissue damage, such as in the intestines. The balance of mTORC1- and/or mTORC2-induced metabolic programs may also tune T reg -cell suppression of effector T-cell responses. For instance, Raptor-deficient T reg cells have increased mTORC2-Akt activity [30] , which can upregulate glycolysis at the expense of mitochondrial metabolism and lead to inappropriate suppression of T H 1 and T FH responses [59] , [60] , [61] . Despite being dispensable for T reg -cell suppressive activity [30] , [61] , mTORC2 can promote T reg -cell trafficking to sites of inflammation and non-lymphoid tissues via upregulating glycolysis or suppressing Foxo1 activity [43] , [62] . Thus, gain of mTORC1 and concomitant loss of mTORC2 activity could reduce T reg -cell trafficking to T H 1 and T H 17 inflammatory sites [63] , [64] , [65] . mTOR may also promote trafficking to sites of T H 2 inflammation by modulating Ccr8 expression and/or CCL22/CCR4-induced chemotaxis [62] , [66] . We, therefore, propose that T reg -cell function is finely tuned by graded nature of mTOR signaling and metabolic programs, which are likely influenced by local environmental signals. This tunable nature of mTOR signaling in T reg cells may offer a therapeutic strategy to modulate T reg -cell responses to selectively alter the conventional T-cell responses in autoimmunity, infectious diseases, and cancer. Mice C57BL/6, CD45.1 + , Cd4 Cre , Foxp3 DTR , Rag1 –/– , Mtor fl , and Tfam fl mice were purchased from The Jackson Laboratory. Foxp3 Cre mice, from Dr. Alexander Rudensky, have been described previously [33] . All genetic models used in this study were on the C57BL/6 background, and both male and female mice were used for quantification and analysis, except for histological analysis where only male mice were used. Mice were generally 4–6-weeks-old unless otherwise indicated. The number of animals in each group are provided in the figures and/or figure legends. All mice were kept in specific pathogen-free conditions within the Animal Resource Center at St. Jude Children’s Research Hospital. The animal protocols were approved by the Institutional Animal Care and Use Committee of St. Jude Children’s Research Hospital. Mixed bone marrow chimeras were generated by adoptive transfer of CD45.1 + bone marrow cells mixed 1:1 with CD45.2 + bone marrow cells from Foxp3 Cre Mtor +/fl or Foxp3 Cre Mtor fl/fl mice into sub-lethally irradiated Rag1 –/– mice as described [30] . For the pT reg cell in vivo maintenance model, CD4 + Foxp3-YFP − CD44 lo CD62L hi naive T cells from the spleens and peripheral lymph nodes of Foxp3 Cre Mtor +/fl or Foxp3 Cre Mtor fl/fl mice were purified on a Synergy or Reflection fluorescence activated cell sorter (Sony Biotechnology). Then, 0.75 × 10 6 cells were transferred via retroorbital injection into sex-matched Rag1 –/– mice. The presence of Foxp3-YFP + T reg cells was evaluated in the mesenteric lymph nodes 4 weeks later [42] . Foxp3 Cre/DTR mosaic mice were treated with DT (50 μg kg −1 ) i.p. three times per week, for a total of four injections. The mice were euthanized, and tissues were harvested for flow cytometry analysis 11 days following the first DT treatment. Sample sizes were chosen based upon previous data generated within the laboratory and were selected to maximize the chance of uncovering statistically significant differences of the mean. No animals were excluded from analysis. Flow cytometry Lymphocytes were harvested form the peripheral lymphoid tissues by manual disruption or the colon lamina propria as previously described [30] , [67] . For surface marker analyses, cells were stained in PBS containing 2% (wt/vol) BSA and the appropriate antibodies. The following fluorescent-conjugate-labeled antibodies, purchased from various commercial sources (Biolegend, BD Biosciences, Thermo Fisher Scientific, and Sony Biotechnology), were used: anti-CD4 (clone RM4-5), anti-CD8 (clone 53-6.7), anti-B220 (clone RA3-6B2), anti-CD62L (clone MEL-14), anti-CD44 (clone IM7), anti-CD95 (clone Jo2), anti-GL7 (clone GL-7), anti-CD279 (PD-1) (Clone J43), and anti-TCRβ (clone H57-597) antibodies. Biotin-conjugated anti-CXCR5 antibody (clone 2G8) and PE-labeled streptavidin from BD Biosciences were used for T FH cell staining. Intracellular staining was performed using the Foxp3/Transcription Factor Staining buffers (Cat #00-5523-00, Thermo Fisher Scientific) per the manufacturer’s instructions. The following antibodies were used: anti-CD152 (CTLA4) (clone UC10-4B9), anti-Foxp3 (clone NRRF-30), anti-RORγt (clone B2D), anti-GATA3 (clone TWAJ), anti-IRF4 (clone 3E4), anti-Helios (clone 22F6), anti-IL-4 (clone 11B11), anti-IL-10 (clone JES5-16E3), anti-IL-13 (clone eBio13A), anti-IFN-γ (clone XMG1.2), anti-IL-17A (clone TC11-18H10.1), anti-human CD25 (clone BC96), anti-human CD45RA (clone HI100), anti-human CD45RO (clone UCHL1), anti-human CD4 (clone A161A1), and anti-human FOXP3 (clone 236 A/E7). For intracellular cytokine staining, total splenocytes were stimulated for 4–5 h with phrobol 12-myristate 13-acetate (PMA) and ionomycin in the presence of monensin (BD Biosciences). Surface and intracellular staining was then performed as above. For active caspase-3 staining, surface molecules were stained before cells were fixed, permeabilized, and stained for intracellular active caspase-3 using the BD Biosciences active caspase-3 apoptosis kit per the manufacturer’s instructions (Cat # 550914). 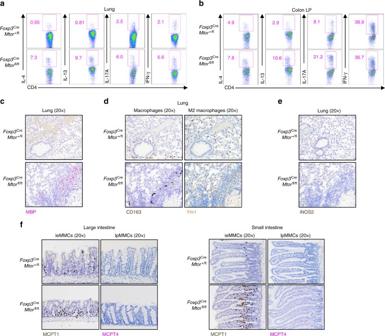Fig. 3 Tregcells require mTOR for the suppression of mucosal TH2 responses.a,bFlow cytometry analysis of cytokine-producing CD4+T cells isolated from the lung (a) or colon lamina propria (LP) (b) ofFoxp3CreMto+/florFoxp3CreMtorfl/flmice.cRepresentative images of major basic protein (MBP) staining for eosinophils in the lung ofFoxp3CreMtor+/flandFoxp3CreMtorfl/flmice.dRepresentative images for M2 macrophages in the lung ofFoxp3CreMtor+/florFoxp3CreMtorfl/flmice by CD163 and Ym1 staining.eRepresentative images for neutrophils, as indicated by inducible nitric oxide synthease 2 (iNOS2) staining, in the lung ofFoxp3CreMtor+/flandFoxp3CreMtorfl/flmice.fRepresentative immunohistochemistry of ieMMCs and lpMMCs in the large intestines (left) and small intestines (right) ofFoxp3CreMtorfl/+orFoxp3CreMtorfl/flmice. Data are representative of four independent experiments (a,b) or three biological replicates per group (c−f). Numbers indicate percentage of cells in gates Staining for mitochondrial dyes (MitoSOX, TMRM, and Mitotracker Deep Red; Thermo Fisher Scientific) was performed as previously described [30] . Histology and immunohistochemistry Tissues were fixed in 10% (vol/vol) neutral buffered formalin solution, embedded in paraffin, section, and stained with hematoxylin and eosin. Blinded samples were analyzed by an experienced pathologist (P.V.) for the presence of lesions indicative of autoimmune disease. For the identification of ieMMCs or lpMMCs, tissue sections from the small intestines and large intestines were respectively stained with primary rat anti-MCPT1 monoclonal antibody (Cat # 14-55303-82, Thermo Fisher Scientific) or goat anti-MCPT4 antibody (LS-B5958, LifeSpan Biosciences) as described previously [37] . GCs were identified by staining with anti-CD3 antibody and peanut agglutinin as described [61] . In vitro T reg -cell suppression assays For analysis of T reg -cell suppression in vitro, CD4 + CD25 hi T reg cells or CD4 + Foxp3-YFP + T reg cells, isolated from the lymphoid organs of the respective Cd4 Cre - or Foxp3 Cre -expressing mice, were co-cultured with naive CD4 + T cells and irradiated splenocytes as antigen presenting cells as previously described [30] . For suppression assays using in vitro activated T reg cells, CD25 hi T reg cells were sorted from the lymphoid organs of C57BL/6 mice, resuspended in complete Click’s medium containing IL-2 (200 U ml −1 ), and activated using anti-CD3 (10 μg ml −1 ) and anti-CD28 (10 μg ml −1 ) antibodies for 3 days in the presence of PP242 (500 nM, Tocris Bioscience) or vehicle control. The live cells were then isolated using Lymphocyte Separation medium and co-cultured with naive CD4 + T cells and irradiated splenocytes for 3 days, and the incorporation of [ 3 H]-thymidine was assessed as described [30] . T reg -cell cultures CD4 + Foxp3-YFP + CD44 lo CD62L hi cT reg cells were purified and activated with anti-CD3 and anti-CD28 antibodies in the presence of recombinant IL-2 for various times in the presence of vehicle, Torin 1 (50 nM) or PP242 (500 nM) before total RNA was harvested using the Qiagen RNeasy micro kit per the manufacturer’s instructions. Alternatively, cT reg cells were stimulated as above for 1–3 days and analyzed by flow cytometry as previously described [43] . For analysis of GATA3 protein expression, CD4 + CD25 + T reg cells were isolated from the mesenteric lymph nodes using the CD25 + T reg -cell enrichment kit (Miltenyi). The cells were then activated with anti-CD3 (5 μg ml −1 ) and anti-CD28 (5 μg ml −1 ) antibodies for 3 days in the presence of various stimuli and/or Torin 1 (50 nM) as indicated in the figure: TGF-β (2 ng ml −1 ), IL-2 (200 U ml −1 ), IL-4 (20 ng ml −1 ), IL-6 (20 ng ml −1 ), and butyrate (125 μM). The expression of GATA3 in Foxp3 + T reg cells was assessed by flow cytometry. Human T reg -cell cultures All human studies were in compliance with the Declaration of Helsinki. Blood donors were recruited by the Blood Donor Center at St. Jude Children’s Research Hospital, where they provided written consent for their discarded blood products to be used for research. This consent form has been reviewed and approved by the Institutional Review Board at St. Jude Children’s Research Hospital. We were provided with apheresis rings containing peripheral blood mononuclear cells (PBMCs) isolated from de-identified donors. Human CD4 + CD25 + CD45RA + CD45RO − naive T reg cells were purified from these human PBMCs, and activated with anti-CD3 (clone OKT3, 5 μg ml −1 ) and anti-CD28 (clone CD28.2, 5 μg ml −1 ) for 3 days in the presence of IL-2 and mTOR inhibitors as above. The expression of human CD25 and human FOXP3 was then analyzed by flow cytometry. Metabolomics CD4 + CD25 hi T reg cells, isolated from lymphoid organs of C57BL/6 mice, were purified and resuspended in complete Click’s medium. Then, 1.3 × 10 6 T reg cells were treated with medium alone or immobilized anti-CD3 antibody (10 μg ml −1 ) and anti-CD28 antibody (10 μg ml −1 ) for 16 h in the presence Torin 1 (50 nM) or vehicle control. Intracellular metabolites, isolated using methanol extraction of two technical replicates, were analyzed using the Ultimate 3000 UHPLC (Dionex) coupled to Q Exactive Plus-Mass spectrometer (QE-MS, Thermo Fisher Scientific) for metabolite profiling. Detailed methods were previously described [68] , except that mobile phase A was replaced with water containing 5 mM ammonium acetate (pH 6.8). Differentially expressed metabolites were identified by Limma (Bioconductor) and the Benjamini-Hochberg method was used to estimate the false discover rate (FDR). MetaboAnalyst was used to analyze range-scale data and provide KEGG pathway analysis of significantly altered metabolic pathways (log 2 = 0.5) ( www.metaboanalyst.ca/ ) [49] . Gene expression analysis For mTOR deletion efficiency in T reg cells, quantitative real-time PCR analysis was performed using Mtor Taqman probes (Thermo Fisher Scientific, Cat #4351372). For detection of Il4 and Il21 , CD4 + Foxp3-YFP – CD44 hi CXCR5 – PD-1 − non-T FH cells or CD4 + Foxp3-YFP – CD44 hi CXCR5 + PD-1 + T FH cells were stimulated for 4 h using plate bound anti-CD3 (5 μg ml −1 ) and anti-CD28 (5 μg ml −1 ) antibodies. Quantitative real-time PCR analysis was performed using SyBR Green Real-Time PCR Master Mix (Thermo Fisher Scientific) and primers for Il4 (Forward 5’-GGTCTCAACCCCCAGCTAGT-3’; Reverse 5’-GCCGATGATCTCTCTCAAGTGAT-3’) and Il21 (Forward 5’-GGACCCTTGTCTGTCTGGTAG-3’; Reverse 5’-TGTGGAGCTGATAGAAGTTCAGG-3’). For microarray analysis, RNA samples from unstimulated cT reg cells or cT reg cells activated in the presence of vehicle, Torin 1, or PP242 for 20 h as indicated above were analyzed with the GeneChip Mouse Gene 2.0 ST Array (Thermo Fisher Scientific). Differentially expressed transcripts in biological triplicate samples were identified by ANOVA (Partek Genomics Suite version 6.5), and the Benjamini-Hochberg method was used to estimate the FDR. GSEA of hallmark pathways in resting vs. activated T reg cells from these microarray samples or published datasets ( GSE55753 [32] or GSE61077 [7] ) was performed as previously described [30] . IRF4 targets were identified from ChIP-seq data [22] deposited in GSE98263 and compared against genes that were differentially expressed in activated cT reg cells treated with or without mTOR inhibitors as above. 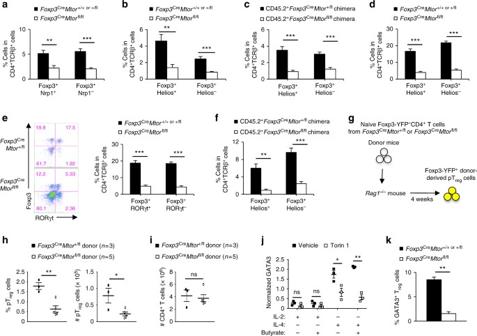Fig. 4 Mucosal tTreg- and pTreg-cell homeostasis is altered in the absence of mTOR.a,bQuantification of the frequencies of Nrp1+and Nrp1–(a) or Helios+and Helios–Tregcells (b) in the lung ofFoxp3CreMtor+/+ or +/flandFoxp3CreMtorfl/flmice, respectively.cQuantification of the frequencies of Helios+and Helios–Tregcells among the CD45.2+CD4+TCRβ+T cells in the lung of mixed bone marrow chimeras.dQuantification of the frequencies of Helios+and Helios–Tregcells in the colon lamina propria ofFoxp3CreMtor+/+ or +/flandFoxp3CreMtorfl/flmice.eFlow cytometry analysis of Foxp3 vs. RORγt expression (left) and quantification of the frequencies of RORγt+and RORγt–Tregcells (right) in the colon lamina propria ofFoxp3CreMtor+/+ or +/flandFoxp3CreMtorfl/flmice.fQuantification of the frequencies of Helios+and Helios–Tregcells among the CD45.2+CD4+TCRβ+T cells in the colon lamina propria of mixed bone marrow chimeras.gExperimental schematic for in vivo pTregmaintenance assay.h,iQuantification of frequency and/or number of donor-derived Foxp3-YFP+pTregcells (h) or total CD4+T cells (i) inRag1–/–mice 4 weeks after adoptive transfer of naive T cells isolated fromFoxp3CreMtor+/flandFoxp3CreMtorfl/flmice.jQuantification of GATA3 expression in Tregcells stimulated under various conditions (with TGF-β and IL-6 included in all the conditions) for 3 days in the presence or absence of Torin 1.kQuantification of GATA3+Tregcells (Foxp3+GATA3+in CD4+TCRβ+) from the colon lamina propria ofFoxp3CreMtor+/+ or +/flandFoxp3CreMtorfl/flmice. Error bars show mean ± s.e.m. *P< 0.05; **P< 0.01; ***P< 0.001; ns, not significant; unpaired, two-tailed Student’st-test. Data are quantified from five (a,b), eight (c), ten (d), eleven (e), seven (f), three or five (h,i; as indicated), three (j), or six (k) biological replicates, compiled from five (a,b), four (c,f), eight (d), nine (e), two (h,i), three (j), or six (k) independent experiments. Numbers indicate percentage of cells in quadrants IRF4 target genes that were differentially expressed in activated cT reg cells treated with mTOR inhibitors were subjected to functional enrichment analysis of metabolism-related pathways, where significance was determined using the Fisher exact test and Benjamini-Hochberg method (FDR < 0.05). Statistics The results in graphs represent the mean ± s.e.m., with the numbers of mice per group and number of experimental replicates indicated in each figure legend. The P -values were calculated with unpaired, two-tailed Student’s t -test assuming equal variance (GraphPad Prism software), where * P < 0.05; ** P < 0.01; *** P < 0.001. No specific randomization methods were used in these studies. 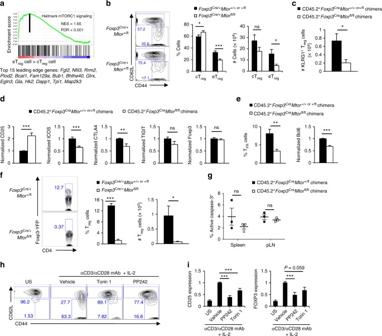Fig. 5 mTOR is essential for eTregcell differentiation.aEnrichment plot of the Hallmark mTORC1 pathway activated in eTregcells compared to cTregcells, identified by gene set enrichment analysis (GSEA). The top 15 enriched genes (position indicated by the vertical black line) are listed below the plot.bFlow cytometry analysis (left) and quantification of frequencies and cell numbers (right) of CD4+Foxp3-YFP+CD44loCD62LhicTregcells and CD4+Foxp3-YFP+CD44hiCD62LloeTregcells inFoxp3Cre/+Mtor+/+or +/flandFoxp3Cre/+Mtorfl/flmosaic mice.cQuantification of the number of KLRG1+Tregcells in the spleen of mixed bone marrow chimeras.dQuantification of CD25, ICOS, CTLA4, TIGIT, and Foxp3 expression in Tregcells from mixed bone marrow chimeras.eQuantification of the frequency of TFRcells (CD4+Foxp3-YFP+CXCR5+PD-1+Tregcells, left) and Bcl6 expression in total Foxp3+Tregcells (right) in mixed bone marrow chimeras.fFlow cytometry analysis (left) and quantification of the frequency and number (right) of Foxp3-YFP+Tregcells in the colon lamina propria ofFoxp3Cre/+Mtor+/+or +/flandFoxp3Cre/+Mtorfl/flmosaic mice.gQuantification of active caspase-3 in CD45.2+CD4+Foxp3-YFP+Tregcells from mixed bone marrow chimeras.hFlow cytometry analysis of CD44 vs. CD62L expression on cTregcells activated under the indicated conditions for 3 days. US: unstimulated.iQuantification of CD25 and FOXP3 expression in human CD4+CD25+CD45RA+CD45RO–naive Tregcells activated for 3 days in the presence or absence of Torin 1 or PP242. Error bars show mean ± s.e.m. *P< 0.05; **P< 0.01; ***P< 0.001; ns, not significant; unpaired, two-tailed Student’st-test. Data are representative of at least six (b), six (f), or three (h) biological replicates per group or are quantified from eleven (b), fifteen (c), seven or eight (d; CD45.2+Foxp3CreMtor+/+ or +/+chimera or CD45.2+Foxp3CreMtor+/+ or +/flmice, respectively; CD25 and Foxp3), ten (d; ICOS, CTLA4, and TIGIT;e), six (f), three (g), or five (i) biological replicates, compiled from seven (b), eight (c), four (d, TIGIT;f), five (d; CD25 and Foxp3), six (d; ICOS and CTLA4;e), or two (g,i) independent experiments. Numbers indicate percentage of cells in gates 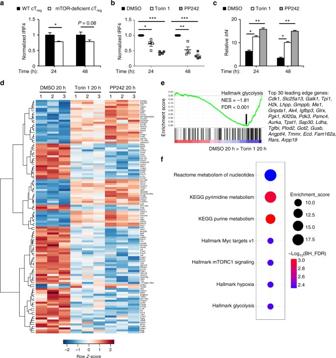Fig. 6 mTOR links activation signals to upregulation of IRF4 expression and downstream targets.aWild-type (WT) and mTOR-deficient CD4+Foxp3-YFP+CD44loCD62LhicTregcells were purified from mixed bone marrow chimeras and activated under the indicated conditions for 24 and 48 h. IRF4 expression was assessed by flow cytometry.bCD4+Foxp3-YFP+CD44loCD62LhicTregcells were purified fromFoxp3Cremice and activated as inain the presence or absence of Torin 1 and PP242. IRF4 expression was assessed by flow cytometry.ccTregcells were purified and activated as inbandIrf4mRNA expression was analyzed by qPCR.dHeat map of IRF4 target genes differentially expressed in resting cTregcells or cTregcells activated in the presence of DMSO, Torin 1, or PP242 for 20 h.eEnrichment plot of the Hallmark glycolysis pathway in cTregcells activated for 20 h in the presence of either Torin 1 or DMSO control, identified by gene set enrichment analysis (GSEA). The top 30 enriched genes (position indicated by the vertical black line) are listed.fFunctional enrichment of the IRF4 target genes shown ind. Error bars show mean ± s.e.m. *P< 0.05; **P< 0.01; ***P< 0.001; ns, not significant; unpaired, two-tailed Student’st-test. Data are representative of three independent experiments (b) or are quantified from five (a) and four (b,c) biological replicates, compiled from two independent experiments (a,c) Investigators were not blinded to samples except where indicated for histological and immunohistochemical analysis. 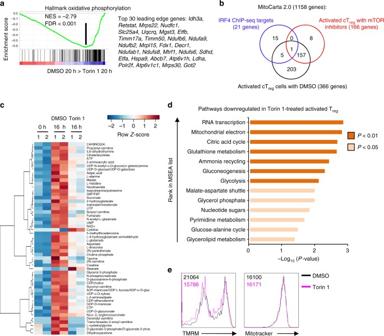Fig. 7 mTOR controls metabolic reprogramming upon Treg-cell activation.aEnrichment plot of the Hallmark oxidative phosphorylation pathway in cTregcells activated for 20 h in the presence of either Torin 1 or DMSO control, identified by gene set enrichment analysis (GSEA). The top 30 enriched genes (position indicated by the vertical black line) are listed.bVenn-diagram depicting mitochondria-related genes (defined in MitoCarta 2.0 database) that are IRF4 targets (blue circle), or differentially expressed in activated cTregcells (vs. unstimulated cells; black circle) or activated cTregcells treated with mTOR inhibitors (vs. those treated with DMSO; red circle). The numbers indicate the shared and independent genes in each category.cHeat map of differentially expressed intracellular metabolites in freshly isolated Tregcells or Tregcells activated for 16 h in the presence of DMSO or Torin 1.dMetabolite set enrichment analysis (MSEA) of KEGG metabolic pathways downregulated in Torin 1-treated activated Tregcells compared to vehicle-treated activated Tregcells.eFlow cytometry of TMRM and Mitotracker staining in Tregcells activated for 20 h in the presence of Torin 1 or vehicle control. Data are representative of three (Mitotracker) or four (TMRM) biological replicates from two (Mitotracker) or three (TMRM) independent experiments (e) 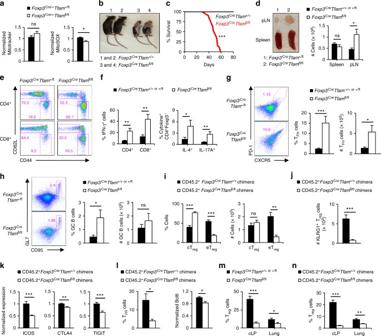Fig. 8 Mitochondrial metabolism is critical for Treg-cell function in vivo.aQuantification of Mitotracker (left) and MitoSOX (right) in Tregcells fromFoxp3Cre/+Tfam+/flandFoxp3Cre/+Tfamfl/flmosaic mice.bImage of 8-week-old mice.cSurvival curve ofFoxp3CreTfam+/+(n= 14) andFoxp3CreTfamfl/flmice (n= 19).dRepresentative image of lymphadenopathy (left) and cell numbers in the spleen and peripheral lymph nodes (pLN) ofFoxp3CreTfam+/flandFoxp3CreTfamfl/flmice.eFlow cytometry analysis of naive and effector/memory CD4+Foxp3-YFP–(depicted as CD4+) or CD8+T cells inFoxp3CreTfam+/flandFoxp3CreTfamfl/flmice.fQuantification of cytokine production by CD4+Foxp3–and CD8+T cells.gFlow cytometry analysis (left) and frequency and number (right) of TFHcells.hFlow cytometry analysis (left) and frequency and number (right) of GC B cells.i,jQuantification of frequencies and numbers of cTregcells and eTregcells (i) or number of KLRG1+Tregcells (j) in the spleen of mixed bone marrow chimeras.kQuantification of ICOS, CTLA4, and TIGIT expression in Tregcells from mixed bone marrow chimeras.lQuantification of the frequency of TFRcells (left) and Bcl6 expression in total Foxp3+Tregcells (right) in mixed bone marrow chimeras.m,nQuantification of frequency of Tregcells in the colon lamina propria and lung ofFoxp3CreTfam+/+ or +/florFoxp3CreTfamfl/flmice (m) or mixed bone marrow chimeras (n). Error bars show mean ± s.e.m. *P< 0.05; **P< 0.01; ***P< 0.001; ns, not significant; unpaired, two-tailed Student’st-test. Data are representative of nine (b,d,e), twelve (g), or ten (h) biological replicates per group, or are quantified from five (a), eight or nine (d,f;Foxp3CreTfamfl/florFoxp3CreTfam+/+ or +/flmice, respectively), twelve (g), ten (h), nine or ten (i−l,n; CD45.2+Foxp3CreTfam+/+chimeras and CD45.2+Foxp3CreTfam+/flchimeras, respectively), five (m, colon), or eight (m, lung) biological replicates per group, compiled from four (a), six (d,f), eight (g), seven (h), four (i−l,n), three (m; colon), or five (m; lung) independent experiments. Numbers indicate percentage of cells in gates Data availability Microarray data that support the findings of this study have been deposited in the Gene Expression Omnibus with the primary accession code GSE104130 . Other data are available from the corresponding author upon request.